Functionally diverse dendritic mRNAs rapidly associate with ribosomes following a novel experience The subcellular localization and translation of messenger RNA (mRNA) supports functional differentiation between cellular compartments. In neuronal dendrites, local translation of mRNA provides a rapid and specific mechanism for synaptic plasticity and memory formation, and might be involved in the pathophysiology of certain brain disorders. Despite the importance of dendritic mRNA translation, little is known about which mRNAs can be translated in dendrites in vivo and when their translation occurs. Here we collect ribosome-bound mRNA from the dendrites of CA1 pyramidal neurons in the adult mouse hippocampus. We find that dendritic mRNA rapidly associates with ribosomes following a novel experience consisting of a contextual fear conditioning trial. High throughput RNA sequencing followed by machine learning classification reveals an unexpected breadth of ribosome-bound dendritic mRNAs, including mRNAs expected to be entirely somatic. Our findings are in agreement with a mechanism of synaptic plasticity that engages the acute local translation of functionally diverse dendritic mRNAs. Subcellular localization of proteins is a highly regulated process that enables different cellular compartments to perform specialized functions. Local translation of messenger RNA (mRNA) is an efficient mechanism for precise subcellular localization of proteins. A striking example of local mRNA translation is found in neurons, where mRNA is trafficked to distal parts of neuronal processes far from their site of transcription in the nucleus. Translation of mRNA in dendrites and axons is performed by locally present ribosomes [1] , [2] , [3] , thereby enabling neurons to develop and modify their synaptic connections with high spatial and temporal resolution [4] . For example, mice with a selective depletion of Camk2a mRNA from neuronal dendrites, but not soma, have synaptic plasticity and memory deficits [5] . Accordingly, dendritic mRNA translation has been proposed as a critical mechanism of memory storage, and has been implicated in the pathophysiology of certain intellectual disability disorders such as Fragile X Syndrome [6] , [7] . Despite the widely accepted importance of dendritic mRNA translation, the full set of genes that encode dendritically localized mRNA, and the conditions that drive local dendritic translation, are currently unknown. Here we present a novel approach based on the expression of epitope-tagged ribosomes in the dendrites of CA1 pyramidal neurons in the mouse hippocampus. This approach enables immunoprecipitation of ribosome-bound dendritic mRNA from the intact brain, thereby resolving two challenges that hampered previous studies. First, because of the inability to physically separate dendrites from intact brain tissue, previous in vivo studies relied on samples containing a mix of dendritic and non-dendritic mRNA without robust means to distinguish these two sources [8] , [9] . Our approach circumvents the challenge of physically separating dendrites from the intact brain, which enabled us to identify 1,890 dendritically localized mRNAs that include many mRNAs assumed to be restricted to the soma. Second, previous genome-wide studies relied on total mRNA samples with unknown ribosome-binding status, making their functional relevance unclear [10] . Here we report that a novel experience increases the association of a large number of dendritic mRNAs with ribosomes, thereby providing strong support for the functional relevance of these dendritic mRNAs. Our findings provide the first in vivo evidence for broad activity-induced changes in ribosome binding of dendritic mRNA. Collecting ribosome-bound mRNA from in vivo dendrites We developed a strategy to collect in vivo dendritic mRNA from adult mouse brains using ribosome immunoprecipitation. Specifically, we created a transgenic mouse in which the Camk2a promoter drives expression of the epitope-tagged ribosomal protein (EGFP-L10a) through the tetracycline transactivator (tTA)–tetO system [11] ( Fig. 1a ). Transgenic mice express EGFP-L10a at high levels in the striatum and in CA1 region of the hippocampus ( Fig. 1b,c ). The interneuron marker Gad1 did not overlap with the EGFP-L10a expression, confirming that within the CA1 region the transgene expression is specific to excitatory pyramidal neurons ( Fig. 1d ). EGFP-L10a expression was seen in the dendrites of CA1 pyramidal neurons ( Fig. 1e ), in agreement with previous reports of dendritic ribosome localization [1] , [2] , [3] . Since previous studies demonstrated the functional incorporation of EGFP-L10a into functional translating ribosomes [12] , [13] , [14] , the observed dendritic expression pattern of EGFP-L10a suggested the possibility of collecting dendritic mRNA by immunoprecipitating dendritically localized green fluorescent protein (GFP)-tagged ribosomes. 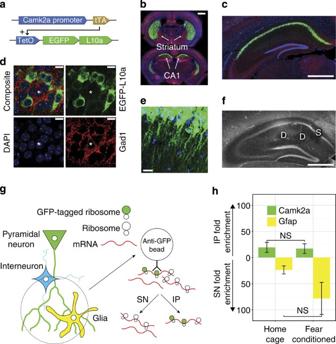Figure 1: A novel method for collectingin vivodendritic mRNA. (a) Camk2a-tTA, TetO-EGFP-L10a double transgenic mice were generated for cell-type-specific expression of EGFP-L10a. (b) EGFP-L10a expression is high in the striatum and dorsal CA1 (Green=EGFP-L10a, Blue=DAPI, Red=Gad1). Scale bar, 1 mm (c) Within the hippocampus the expression of EGFP-L10a is limited to the CA1 region. Scale bar, 0.5 mm (d) Within the CA1 region the expression of EGFP-L10a is restricted to excitatory pyramidal neurons (Green=EGFP-L10a, Blue=DAPI, Red=Gad1 and asterisk indicates Gad1-positive cell). Scale bars, 10 μm (e) EGFP-L10a is present in the dendrites of CA1 pyramidal neurons. Scale bar, 20 μm (f) Representative example of the location of somatic (S) and dendritic (D) punches in the CA1. Scale bar, 0.5 mm (g) Diagram showing the approach used for collecting ribosome-bound mRNA fromin vivodendrites. The immunoprecipitate (IP) will contain mRNA bound to ribosomes in CA1 pyramidal neuron dendrites while the supernatant (SN) will contain mRNA from other sources. (h) qPCR analysis of dendritic mRNA samples from home cage (n=6) and contextual fear conditioned (n=5) mice confirms the expected IP enrichment of Camk2a and SN enrichment of the astrocyte-specific gene Gfap. Error bars represent s.e.m. NS, not significant. Figure 1: A novel method for collecting in vivo dendritic mRNA. ( a ) Camk2a-tTA, TetO-EGFP-L10a double transgenic mice were generated for cell-type-specific expression of EGFP-L10a. ( b ) EGFP-L10a expression is high in the striatum and dorsal CA1 (Green=EGFP-L10a, Blue=DAPI, Red=Gad1). Scale bar, 1 mm ( c ) Within the hippocampus the expression of EGFP-L10a is limited to the CA1 region. Scale bar, 0.5 mm ( d ) Within the CA1 region the expression of EGFP-L10a is restricted to excitatory pyramidal neurons (Green=EGFP-L10a, Blue=DAPI, Red=Gad1 and asterisk indicates Gad1-positive cell). Scale bars, 10 μm ( e ) EGFP-L10a is present in the dendrites of CA1 pyramidal neurons. Scale bar, 20 μm ( f ) Representative example of the location of somatic (S) and dendritic (D) punches in the CA1. Scale bar, 0.5 mm ( g ) Diagram showing the approach used for collecting ribosome-bound mRNA from in vivo dendrites. The immunoprecipitate (IP) will contain mRNA bound to ribosomes in CA1 pyramidal neuron dendrites while the supernatant (SN) will contain mRNA from other sources. ( h ) qPCR analysis of dendritic mRNA samples from home cage ( n =6) and contextual fear conditioned ( n =5) mice confirms the expected IP enrichment of Camk2a and SN enrichment of the astrocyte-specific gene Gfap. Error bars represent s.e.m. NS, not significant. Full size image As previous in vitro studies found that ribosome association of dendritic mRNA changes after neuronal activation [15] , [16] , [17] , [18] , [19] , [20] , [21] , we sought to determine if this also occurs in vivo . To detect activity-induced changes, we collected ribosome-bound mRNA from mice in a resting state and from mice subjected to a novel experience. Specifically, we collected CA1 tissue punches from transgenic mice either resting in their home cage or immediately after a 500-s contextual fear conditioning trial. Expression of EGFP-L10a did not affect contextual fear conditioning behaviour ( Supplementary Fig. 1a ), and EGFP-L10a expression was similar between home cage and contextual fear conditioned mice ( Supplementary Fig. 1b ). Tissue punches were placed in either the CA1 layer containing the dendrites of pyramidal neurons (dendritic punches) or in the CA1 layer containing the soma of pyramidal neurons (somatic punches) ( Fig. 1f ). Accurately placed dendritic and somatic punches from individual mice were pooled and subjected to an immunoprecipitation protocol optimized for low background ( Supplementary Fig. 1c–f ). This enabled us to obtain immunoprecipitate (IP) fractions containing either dendritic or somatic mRNA bound to GFP-tagged ribosomes ( Fig. 1g ). The mRNA in both the IP and the supernatant (SN) fractions was isolated for further analysis. In agreement with the predicted presence of dendritic mRNA in the IP of dendritic punches, quantitative PCR (qPCR) analysis showed enrichment of the known dendritic mRNA Camk2a in the IP of home cage and contextual fear conditioned mice, while the glial gene Gfap was enriched in the SN of both groups, illustrating the specificity of the immunoprecipitation ( Fig. 1h ). Dendritic mRNAs rapidly bind ribosomes upon novel experience We used high throughput RNA sequencing (RNA-Seq) to perform genome-wide characterization of dendritic and somatic mRNA bound to GFP-tagged ribosomes ( Supplementary Table 1 ). Analysis of sequencing read distribution revealed that a smaller number of sequencing reads aligned to the 3′ untranslated regions (3′UTR) in IP samples compared with SN samples ( Fig. 2a ). Further characterization of this 3′UTR depletion revealed a decrease in IP read coverage ~200 nucleotides after the stop codon with a concomitant increase in SN read coverage ( Fig. 2b ). This loss of 3′UTR reads in the IP can be explained by RNA fragmentation that occurred during the tissue processing steps and immunoprecipitation. Because ribosomes bind to the 5′UTR and coding sequence (CDS) of transcripts and fall off at the stop codon preceding the 3′ UTR, random RNA fragmentation would produce distal 3′UTR fragments that are not associated with GFP-tagged ribosomes and therefore end up in the SN ( Fig. 2c ). The depletion of 3′UTR reads observed in the IP samples therefore supports the predicted ribosome-bound state of the mRNAs in the IP samples. 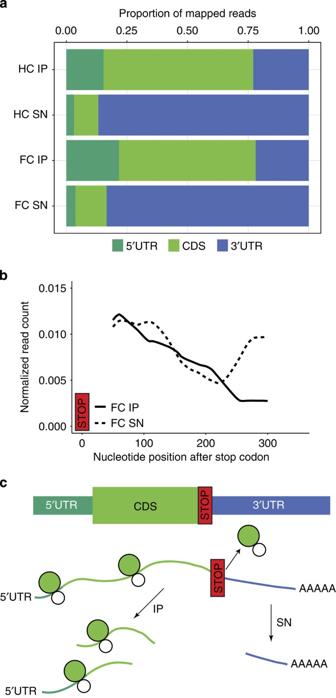Figure 2: RNA-Seq analysis confirms the ribosome-bound status of immunoprecipitated mRNA. (a) Dendritic immunoprecipitate (IP) samples had a smaller proportion of RNA-Seq reads mapping to the 3′UTR as compared with dendritic supernatant (SN) samples (CDS, coding sequence; FC, contextual fear conditioning; HC, home cage; UTR, untranslated region). (b) Depletion of 3′UTR reads in the dendritic IP started ~200 nucleotides after the stop codon as indicated by a decline in read coverage in the IP and a concomitant increase in read coverage in the SN. Read coverage was calculated for a set of genes that within the CA1 are only expressed in pyramidal neurons (+pyr genes, see Methods for details). (c) Diagram explaining how the depletion of 3′UTR reads in the IP confirms the expected ribosome-bound status of immunoprecipitated mRNA. As ribosomes bind to the 5′UTR and CDS of transcripts, random fragmenting of RNA would cause distal portions of the 3′UTR to remain in the SN. Figure 2: RNA-Seq analysis confirms the ribosome-bound status of immunoprecipitated mRNA. ( a ) Dendritic immunoprecipitate (IP) samples had a smaller proportion of RNA-Seq reads mapping to the 3′UTR as compared with dendritic supernatant (SN) samples (CDS, coding sequence; FC, contextual fear conditioning; HC, home cage; UTR, untranslated region). ( b ) Depletion of 3′UTR reads in the dendritic IP started ~200 nucleotides after the stop codon as indicated by a decline in read coverage in the IP and a concomitant increase in read coverage in the SN. Read coverage was calculated for a set of genes that within the CA1 are only expressed in pyramidal neurons (+pyr genes, see Methods for details). ( c ) Diagram explaining how the depletion of 3′UTR reads in the IP confirms the expected ribosome-bound status of immunoprecipitated mRNA. As ribosomes bind to the 5′UTR and CDS of transcripts, random fragmenting of RNA would cause distal portions of the 3′UTR to remain in the SN. Full size image The RNA-Seq data enabled us to further test the expected enrichment of dendritic mRNA in the IP samples by looking at a larger set of control genes than would be practical with qPCR analysis. For this, we used a positive-control set of 74 genes that within the CA1 are exclusively expressed in the pyramidal neurons (+pyr; for example, Camk2a and Ddn ; Fig. 3a ), and a negative-control set of 124 genes that within the CA1 are exclusively expressed outside of the pyramidal neurons (−pyr; for example Gad1 and Gfap ; Fig. 3b ). The +pyr and −pyr lists were created by manually curating the in situ images of 1,238 genes available through the Allen Mouse Brain Atlas ( Supplementary Data 1 ). The levels of +pyr and −pyr mRNAs were quantified as Fragments Per Kilobase of gene length per Million mapped reads (FPKM) values (see Methods for details). Because of the decreased 3′UTR read coverage starting ~200 nucleotides after the stop codon in the IP samples ( Fig. 2b ), we calculated mRNA levels using a FPKM value based on the RNA-Seq reads that mapped upstream of 200 nucleotides after the stop codon (FPKM CDS(+) ; see Methods for details). By calculating the ratio of IP FPKM CDS(+) to SN FPKM CDS(+) , we determined the level of IP or SN enrichment for each +pyr gene and each −pyr gene. In agreement with the Camk2a and Gfap qPCR results ( Fig. 1h ), +pyr genes were on an average enriched in the IP, while −pyr genes were on an average enriched in the SN ( Fig. 3c ). Because the +pyr and −pyr gene lists were obtained independently from our RNA-Seq expression data, the observed IP enrichment of +pyr genes provides a strong confirmation of the expected enrichment of dendritic mRNA in the IP samples. 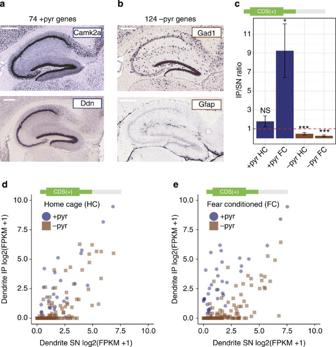Figure 3: Fear conditioning increases ribosome binding to dendritic mRNA. (a) Examples of +pyr control genes with exclusive expression only in CA1 pyramidal cells. Scale bar, 0.4 mm (b) Examples of –pyr control genes with expression only outside of CA1 pyramidal cells (aandb: images from Allen Mouse Brain Atlas25). Scale bar, 0.4 mm (c) In agreement with the enrichment of dendritic mRNA in the IP of dendritic punches, +pyr genes were on an average enriched in the IP (IP/SN ratio>1), while –pyr genes were on an average enriched in the SN (IP/SN ratio<1; CDS(+) FPKM values calculated from RNA-Seq data were used to calculate IP/SN ratios; red dashed line indicates IP/SN=1; error bars represent s.e.m; Wilcoxon signed rank tests versus IP/SN=1 were performed for each group: NS=not significant, *=P<0.05, ***=P<0.0001). (d) Limited enrichment of dendritic mRNA in the home cage IP as indicated by a partial overlap between +pyr and –pyr genes in a scatterplot of IP and SN expression values (CDS(+) log2(FPKM+1) values calculated from the home cage dendritic RNA-Seq data were used to obtain expression values). (e) Fear conditioning increased enrichment of dendritic mRNA as indicated by increased separation between +pyr and –pyr genes (scatterplot generated similar to (d) except contextual fear conditioning dendritic RNA-Seq data were used). The increased enrichment of dendritic mRNA indicates increased ribosome binding of dendritic mRNA as a result of fear conditioning. Figure 3: Fear conditioning increases ribosome binding to dendritic mRNA. ( a ) Examples of +pyr control genes with exclusive expression only in CA1 pyramidal cells. Scale bar, 0.4 mm ( b ) Examples of –pyr control genes with expression only outside of CA1 pyramidal cells ( a and b : images from Allen Mouse Brain Atlas [25] ). Scale bar, 0.4 mm ( c ) In agreement with the enrichment of dendritic mRNA in the IP of dendritic punches, +pyr genes were on an average enriched in the IP (IP/SN ratio>1), while –pyr genes were on an average enriched in the SN (IP/SN ratio<1; CDS(+) FPKM values calculated from RNA-Seq data were used to calculate IP/SN ratios; red dashed line indicates IP/SN=1; error bars represent s.e.m; Wilcoxon signed rank tests versus IP/SN=1 were performed for each group: NS=not significant, *= P <0.05, ***= P <0.0001). ( d ) Limited enrichment of dendritic mRNA in the home cage IP as indicated by a partial overlap between +pyr and –pyr genes in a scatterplot of IP and SN expression values (CDS(+) log2(FPKM+1) values calculated from the home cage dendritic RNA-Seq data were used to obtain expression values). ( e ) Fear conditioning increased enrichment of dendritic mRNA as indicated by increased separation between +pyr and –pyr genes (scatterplot generated similar to ( d ) except contextual fear conditioning dendritic RNA-Seq data were used). The increased enrichment of dendritic mRNA indicates increased ribosome binding of dendritic mRNA as a result of fear conditioning. Full size image Though the qPCR and RNA-Seq data of both the home cage and contextual fear conditioned samples were in agreement with an enrichment of dendritic mRNA in the IP ( Figs 1h and 3c ), this enrichment appeared to be stronger after contextual fear conditioning (see +pyr genes in Fig. 3c ). To confirm that the IP samples from contextual fear conditioned mice differed from the IP samples of home cage mice, we performed clustering analysis of all the RNA-Seq data obtained from home cage and contextual fear conditioned IP samples. This revealed that the contextual fear conditioned IP samples clustered separately from the home cage IP samples ( Supplementary Fig. 2 ). Furthermore, scatterplots of all the individual +pyr and –pyr genes showed a better separation between +pyr and −pyr genes after contextual fear conditioning compared with home cage ( Fig. 3d,e ), in agreement with a higher IP enrichment of dendritic mRNA after contextual fear conditioning. The higher IP enrichment of dendritic mRNA after contextual fear conditioning could not have been caused by increased gene transcription, as the 500 s duration of the contextual fear conditioning trial did not provide sufficient time for mRNA to be transcribed, processed and transported to dendrites [22] , [23] . The increased enrichment of dendritic mRNA in the IP after contextual fear conditioning therefore reflects changes in the ribosome binding of mRNAs that were already present in the dendrites, revealing that dendritic mRNAs rapidly associate with ribosomes following a novel experience. Machine learning classification predicts new dendritic mRNAs Given the broad enrichment of +pyr genes in the dendrite IP after fear conditioning ( Fig. 3c,e ), we anticipated that the underlying RNA-Seq data could be used for the genome-wide discovery of dendritic mRNAs. We applied a supervised machine learning algorithm to our contextual fear conditioning dendrite RNA-Seq data, thereby enabling discovery of novel dendritic mRNAs. Specifically, we employed a linear support vector machine (SVM) algorithm using the +pyr and −pyr genes as training sets with four FPKM values per gene (FPKM CDS(+) for IP and SN, and FPKM 3′UTR(−) for IP and SN; see Methods for details). The FPKM CDS(+) was calculated as described earlier, while the FPKM 3′UTR(−) was calculated using the RNA-Seq reads that mapped to the 3′UTR region downstream of 200 nucleotides after the stop codon. The location of the CDS(+)/3′UTR(−) split at 200 nucleotides after the stop codon was based on the observed switch in 3′UTR coverage at this location ( Fig. 2b ), and was further validated by performing separate rounds of machine learning classification using alternative CDS(+)/3′UTR(−) splits ( Supplementary Fig. 3a,c ). Our machine learning classification generated a list of 1,890 unique mRNAs predicted to be bound to ribosomes in CA1 pyramidal neuron dendrites after fear conditioning (false positive rate: 0.056; false negative rate: 0.094; Supplementary Data 2 ). For genes with a high FPKM CDS(+) (>1), the classification was largely based on the FPKM CDS(+) ( Fig. 4a ). In contrast, we found that for genes with a low FPKM CDS(+) (<1) the classification was less based on the FPKM CDS(+) ( Fig. 4b ), but instead was more based on the FPKM 3′UTR(−) ( Fig. 4c ). This indicated that including the FPKM 3′UTR(−) in our machine learning algorithm enabled a more accurate classification for a subset of genes with lower expression values ( Supplementary Fig. 3e–i ). Machine learning produced poor classification results for the RNA-Seq data generated from home cage dendritic punches, in accordance with the incomplete separation between +pyr and −pyr genes ( Fig. 3d ; Supplementary Fig. 3b,d ). 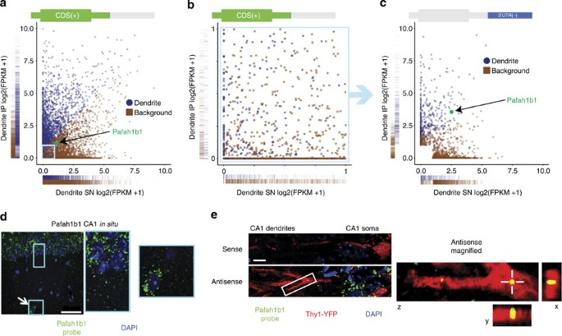Figure 4: Machine learning prediction of dendritically localized mRNAs. (a) Classification of dendritic mRNAs by machine learning analysis of contextual fear conditioning dendritic RNA-Seq data (blue=dendritic, brown=background). One-dimensional density (rug) plots on the x and y axes show that mRNAs classified as dendritic have in general higher IP FPKMCDS(+)values and lower SN FPKMCDS(+)values when compared with mRNAs classified as background. One of the exceptions, Pafah1b1, is highlighted in green. Pafah1b1 is classified as dendritic despite having IP and SN FPKMCDS(+)values more similar to mRNAs classified as background. The light blue box indicates the area magnified inFig. 4b. (b) Dendritic classification of mRNAs with low FPKMCDS(+)values (both IP and SN<1) is not based on FPKMCDS(+)values as indicated by the intermixing of mRNAs classified as dendritic and background. (c) The same mRNAs as shown inFig. 4b, this time plotted using the FPKM3′UTR(−)values. Pafah1b1 (green) is an example of an mRNA classified as dendritic mainly based on the FPKM3′UTR(−)values. Also seeSupplementary Fig. 3e–i. (d) Pafah1b1in situusing a FISH probe shows Pafah1b1 expression in the soma of pyramidal neurons (rectangular box) and an interneuron (square box with arrow) in the CA1 region. Scale bar, 50 μm. (e)In situhybridization of Pafah1b1 mRNA in Thy1–YFP transgenic tissue shows punctate labelling within dendrites, which is absent when using a sense probe (green=Pafah1b1 probe, red=Thy1–YFP and blue=DAPI). Scale bar, 10 μm. On the right is a magnified view of the area indicated by the white box showing a Pafah1b1 mRNA puncta located within a YFP-labelled dendrite (crosshair in z view marks same puncta shown in x and y views). Figure 4: Machine learning prediction of dendritically localized mRNAs. ( a ) Classification of dendritic mRNAs by machine learning analysis of contextual fear conditioning dendritic RNA-Seq data (blue=dendritic, brown=background). One-dimensional density (rug) plots on the x and y axes show that mRNAs classified as dendritic have in general higher IP FPKM CDS(+) values and lower SN FPKM CDS(+) values when compared with mRNAs classified as background. One of the exceptions, Pafah1b1, is highlighted in green. Pafah1b1 is classified as dendritic despite having IP and SN FPKM CDS(+) values more similar to mRNAs classified as background. The light blue box indicates the area magnified in Fig. 4b . ( b ) Dendritic classification of mRNAs with low FPKM CDS(+) values (both IP and SN<1) is not based on FPKM CDS(+) values as indicated by the intermixing of mRNAs classified as dendritic and background. ( c ) The same mRNAs as shown in Fig. 4b , this time plotted using the FPKM 3′UTR(−) values. Pafah1b1 (green) is an example of an mRNA classified as dendritic mainly based on the FPKM 3′UTR(−) values. Also see Supplementary Fig. 3e–i . ( d ) Pafah1b1 in situ using a FISH probe shows Pafah1b1 expression in the soma of pyramidal neurons (rectangular box) and an interneuron (square box with arrow) in the CA1 region. Scale bar, 50 μm. ( e ) In situ hybridization of Pafah1b1 mRNA in Thy1–YFP transgenic tissue shows punctate labelling within dendrites, which is absent when using a sense probe (green=Pafah1b1 probe, red=Thy1–YFP and blue=DAPI). Scale bar, 10 μm. On the right is a magnified view of the area indicated by the white box showing a Pafah1b1 mRNA puncta located within a YFP-labelled dendrite (crosshair in z view marks same puncta shown in x and y views). Full size image As a first validation of our machine learning results, we tested the predicted dendritic presence of Pafah1b1 mRNA using fluorescent in situ hybridization (FISH). We chose Pafah1b1 for several reasons. First, Pafah1b1 is an example of a gene classified primarily through its FPKM 3′UTR(−) ( Fig. 4a,c ), and confirming its dendritic presence would therefore further validate the use of separate FPKM CDS(+) and FPKM 3′UTR(−) values in our machine learning algorithm. Second, Pafah1b1 was previously detected in a RNA-Seq analysis of dendrite-containing CA1 neuropil, but it was not classified as a dendritic mRNA because of its known presence in interneurons that surround the dendrites of CA1 pyramidal neurons [8] . Confirming the dendritic presence of Pafah1b1 mRNA would therefore exemplify the benefit of our strategy for unbiased discovery of dendritic mRNAs. Third, mutations in the Pafah1b1 gene, also known as Lis1 ( lissencephaly-1 ), are associated with autism and intellectual disability, and accordingly the Pafah1b1 protein is required for normal dendritic spine plasticity [24] . Demonstrating the dendritic presence of Pafah1b1 mRNA would contribute to the mechanistic understanding of Pafah1b1 ’s role in synaptic plasticity and neurodevelopment. FISH analysis confirmed the expression of Pafah1b1 in both excitatory neurons and interneurons within the CA1 dendritic layer, consistent with in situ images from the Allen Mouse Brain Atlas [25] ( Fig. 4d ). FISH performed on a Thy1–yellow fluorescent protein (YFP) mouse brain was used for the detection of Pafah1b1 mRNA within sparsely labelled CA1 pyramidal neurons [26] . This revealed punctate Pafah1b1 mRNA labelling within dendrites of CA1 excitatory neurons, thereby confirming the dendritic presence of Pafah1b1 mRNA as predicted by our machine learning analysis ( Fig. 4e ). Expected soma-restricted mRNAs can localize in dendrites We used Gene Ontology (GO) analysis to gain a more comprehensive understanding of the types of mRNAs that can localize in dendrites. To enable a comparison between predicted dendritic and somatic mRNAs, we employed machine learning classification to obtain a list of 2,903 unique mRNAs predicted to be bound to ribosomes in CA1 pyramidal neuron soma after contextual fear conditioning (false positive rate: 0.216; false negative rate: 0.133; Fig. 5a and Supplementary Fig. 4a–c ; Supplementary Data 3 ). For the GO analysis we used the top 75th percentile in the contextual fear conditioning dendritic and somatic mRNA lists to focus on the more highly enriched genes. As expected, the dendritic and somatic lists showed different enrichment profiles (selected categories in Fig. 5b , top 20 categories in Supplementary Fig. 4d ). Genes involved in translation and the cytoskeleton were the most enriched in the contextual fear conditioning dendritic list, in agreement with previous reports and suggesting the importance of increased local translation and cytoskeleton remodelling in dendrites shortly after neuronal activation [27] , [28] . Unexpectedly, the dendritic list also showed enrichment in mRNAs encoding proteins known for their functions inside the nucleus, such as those involved in chromosome organization and transcriptional regulation ( Fig. 5b ). While in vitro studies have observed the dendritic localization of transcription factor mRNA [29] , a previous in vivo study had to exclude mRNAs encoding proteins with nuclear functions from the analysis due to potential interneuron or glia origins [8] . The list of dendritic mRNA predicted by our unbiased classification included several gene families with well-known nuclear functions. These included H4 histones, which are part of the core histone complex [30] , and members of the mediator complex, which is an important regulator of gene transcription [31] . Out of the seven H4 histone mRNAs detected in our RNA-Seq data, three were predicted to be localized in dendrites, and out of the 21 detected mediator mRNAs, seven were predicted to be localized in dendrites ( Fig. 5b ). 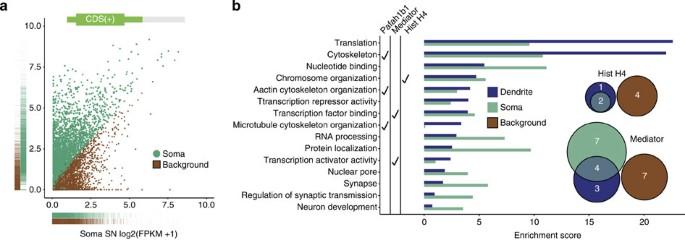Figure 5: Gene ontology enrichment analysis reveals unexpected classes of ribosome-bound dendritic transcripts. (a) Classification of somatic mRNAs by machine learning analysis of contextual fear conditioning somatic RNA-Seq data (green=somatic and brown=background). (b) Gene ontology (GO) enrichment analysis of dendritic and somatic mRNAs. In agreement with previous studies27,28, dendritic mRNAs were highly enriched in translation and cytoskeleton GO categories. Unexpected GO categories with dendritic mRNA enrichment included chromosome organization and transcription factor binding. GO categories that include the Pafah1b1 gene, mediator genes and H4 histone genes are indicated. Venn diagram insets show the number of unique histone H4 and mediator mRNAs that were detected in the RNA-Seq data as well as their classifications. Also seeSupplementary Fig. 4. Figure 5: Gene ontology enrichment analysis reveals unexpected classes of ribosome-bound dendritic transcripts. ( a ) Classification of somatic mRNAs by machine learning analysis of contextual fear conditioning somatic RNA-Seq data (green=somatic and brown=background). ( b ) Gene ontology (GO) enrichment analysis of dendritic and somatic mRNAs. In agreement with previous studies [27] , [28] , dendritic mRNAs were highly enriched in translation and cytoskeleton GO categories. Unexpected GO categories with dendritic mRNA enrichment included chromosome organization and transcription factor binding. GO categories that include the Pafah1b1 gene, mediator genes and H4 histone genes are indicated. Venn diagram insets show the number of unique histone H4 and mediator mRNAs that were detected in the RNA-Seq data as well as their classifications. Also see Supplementary Fig. 4 . Full size image To test the predicted dendritic presence of mRNAs encoding H4 histones and mediator proteins, we used FISH and immunohistochemisty (IHC) to image the subcellular localization of one member of the H4 histone gene family ( Hist1h4j ) and one member of the mediator gene family ( Med8 ). FISH using an antisense probe specific for Hist1h4j confirmed the presence of Hist1h4j mRNA within the dendrites of Thy1–YFP-labelled CA1 pyramidal neurons ( Fig. 6a ). IHC using a histone H4-specific antibody resulted in the expected punctate labelling within the nuclei of CA1 pyramidal neurons, but in addition also resulted in punctate labelling within dendrites ( Fig. 6b ). The histone H4 antibody produced a similar punctate staining pattern in the nuclei and dendrites of Thy1–YFP-labelled pyramidal neurons in the cortex ( Supplementary Fig. 5a ). FISH and IHC analysis of Med8 generated results similar to the Hist1h4j results. As predicted by our machine learning results, Med8 mRNA was detected within the dendrites of CA1 pyramidal neurons ( Fig. 7a ). IHC with a Med8-specific antibody resulted in the expected punctate labelling within nuclei, as well as punctate labelling within CA1 and cortical dendrites ( Fig. 7b ; Supplementary Fig. 5b ). The FISH and IHC data confirm that our list of 1,890 putative ribosome-bound dendritic transcripts can be used to predict the dendritic localization of specific mRNAs and their protein products, even when these proteins were previously assumed to be exclusively localized within the nucleus. 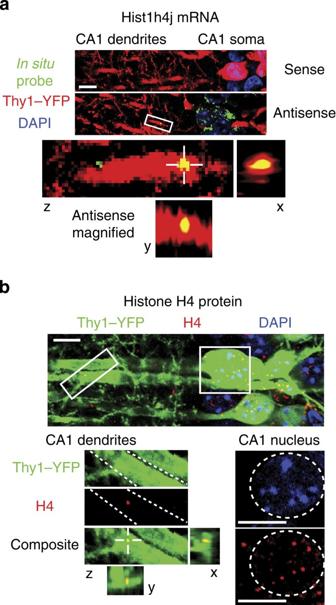Figure 6: Dendritic localization of mRNA and protein encoded by the chromatin-associated gene Hist1h4j. (a)In situhybridization for Hist1h4j shows puncta within YFP-labelled dendrites with the antisense probe, but not with the sense probe (green=Hist1h4j probe, red=YFP and blue=DAPI). The bottom panels show magnified views of the area indicated by the white box. Views from all three planes show colocalization between Hist1h4j mRNA and the YFP-labelled dendrite. (b) Histone H4 IHC results in dendritically localized puncta (green=Thy1–YFP, red=histone H4 and blue=DAPI). Magnified dendritic and somatic areas are indicated with white boxes. Dashed white lines in the magnified dendritic image outline a single dendrite. Views from all three planes show colocalization between histone H4 protein and the dendrite. A dashed white circle in the magnified somatic image outlines a nucleus with the expected presence of histone H4 protein. Scale bars, 10 μm. Figure 6: Dendritic localization of mRNA and protein encoded by the chromatin-associated gene Hist1h4j. ( a ) In situ hybridization for Hist1h4j shows puncta within YFP-labelled dendrites with the antisense probe, but not with the sense probe (green=Hist1h4j probe, red=YFP and blue=DAPI). The bottom panels show magnified views of the area indicated by the white box. Views from all three planes show colocalization between Hist1h4j mRNA and the YFP-labelled dendrite. ( b ) Histone H4 IHC results in dendritically localized puncta (green=Thy1–YFP, red=histone H4 and blue=DAPI). Magnified dendritic and somatic areas are indicated with white boxes. Dashed white lines in the magnified dendritic image outline a single dendrite. Views from all three planes show colocalization between histone H4 protein and the dendrite. A dashed white circle in the magnified somatic image outlines a nucleus with the expected presence of histone H4 protein. Scale bars, 10 μm. 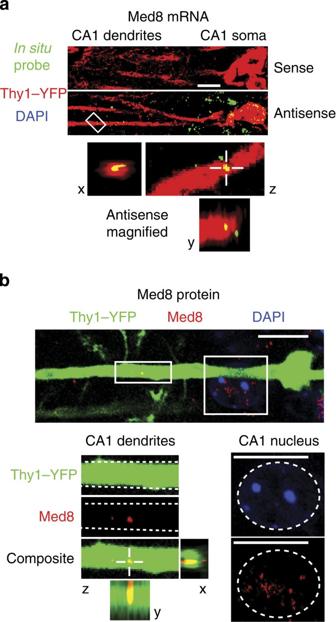Figure 7: Dendritic localization of mRNA and protein encoded by the transcription-associated gene Med8. (a)In situhybridization for Med8 shows puncta within YFP-labelled dendrites with the antisense probe, but not with the sense probe (green=Med8 probe, red=YFP and blue=DAPI). The bottom panels show magnified views of the area indicated by the white box. Views from all three planes show colocalization between Med8 mRNA and the YFP-labelled dendrite. (b) Med8 IHC results in dendritically localized puncta (green=Thy1–YFP, red=Med8 and blue=DAPI). Magnified dendritic and somatic areas are indicated with white boxes. Dashed white lines in the magnified dendritic image outline a single dendrite. Views from all three planes show colocalization between Med8 protein and the dendrite. A dashed white circle in the magnified somatic image outlines a nucleus with the expected presence of Med8 protein. Scale bars, 10 μm. Full size image Figure 7: Dendritic localization of mRNA and protein encoded by the transcription-associated gene Med8. ( a ) In situ hybridization for Med8 shows puncta within YFP-labelled dendrites with the antisense probe, but not with the sense probe (green=Med8 probe, red=YFP and blue=DAPI). The bottom panels show magnified views of the area indicated by the white box. Views from all three planes show colocalization between Med8 mRNA and the YFP-labelled dendrite. ( b ) Med8 IHC results in dendritically localized puncta (green=Thy1–YFP, red=Med8 and blue=DAPI). Magnified dendritic and somatic areas are indicated with white boxes. Dashed white lines in the magnified dendritic image outline a single dendrite. Views from all three planes show colocalization between Med8 protein and the dendrite. A dashed white circle in the magnified somatic image outlines a nucleus with the expected presence of Med8 protein. Scale bars, 10 μm. Full size image We have developed and applied a novel method for collecting ribosome-bound mRNA from in vivo dendrites. The genome-wide analysis of this mRNA revealed two important properties of in vivo dendritically localized mRNA. First, dendritic mRNA encodes proteins with a large variety of functions, including proteins whose only known functions are in the nucleus. Second, many dendritic mRNAs rapidly associate with ribosomes upon a novel experience. Our method for collecting ribosome-bound dendritic mRNA circumvents the long-standing challenge of physically separating dendrites from intact brain tissue. Because of this challenge, previous studies used either cultured neurons [32] , [33] or, when using brain tissue [8] , [9] , could not predict the dendritic localization of mRNAs that are also present in cells immediately adjacent to dendrites. For example, 848 out of the 1,890 mRNAs in our dendritic list were also detected in a previous study using neuropil mRNA, but they had to be excluded from the final analysis due to potential non-dendritic sources [8] (for example, Pafah1b1 ; Fig. 4d,e ; Supplementary Fig. 6 ; Supplementary Data 4 ). Out of these 848 mRNAs, 198 mRNAs were excluded because they encode proteins with nuclear functions [8] . Our confirmation of the dendritic presence of Hist1h4j and Med8 mRNA, both encoding proteins with a nuclear function, illustrates the benefit of our unbiased classification. Classification was achieved in our study with a supervised machine learning algorithm trained to perform with the highest possible sensitivity and specificity (see Supplementary Fig. 3c ). This resulted in a list of 1,890 mRNAs that are predicted to be ribosome bound in dendrites shortly after a novel experience. It should be noted that the estimated false positive rate for this list (0.056) suggests that ~106 mRNAs out of our list of 1,890 mRNAs could represent mRNAs that were not bound to ribosomes in dendrites, but instead might have been located in cells that surround the dendrites (such as interneurons, glia and epithelial cells). Such mRNAs could have bound nonspecifically to the beads during the immunoprecipitation. Though it is impossible to completely eliminate this nonspecific binding, it was greatly reduced with our optimized immunoprecipitation protocol (see Supplementary Fig. 1c–f ). The impact of any remaining nonspecific binding was reduced by sequencing both the IP and SN fractions. This enabled us to distinguish mRNAs with relatively high IP/SN ratios from mRNAs with relatively low IP/SN ratios. Higher IP/SN ratios are more likely caused by specific binding of GFP-tagged ribosomes to the beads. Accordingly, after fear conditioning almost all negative-control genes (−pyr) had lower IP/SN ratios compared with all positive-control genes (+pyr; see Fig. 3e ). This enabled us to use the +pyr and –pyr genes as training sets for a supervised machine learning algorithm, which determined the optimal use of our genome-wide IP and SN expression values for generating a list of predicted dendritic mRNAs. Despite our precautions to reduce the occurrence and impact of nonspecific mRNA binding during the immunoprecipitation, we can not exclude the possibility that a fraction of the 1,890 predicted dendritic mRNAs are actually non-dendritic. Further in-situ hybridization experiments will therefore be useful to verify the subcellular localization of predicted dendritic mRNAs. Our list of predicted dendritically localized transcripts was obtained from ribosome-bound mRNA samples. This is an important advance compared with previous dendritic mRNA studies, which relied on total mRNA that might or might not have been associated with ribosomes. Detection of a dendritic mRNA with an unknown ribosome association status leaves open the possibility that the mRNA is never translated and is merely a nonfunctional by-product of mRNA diffusion from the soma. Though the ribosome-bound status of the mRNA samples analyzed in our study make it unlikely that these mRNAs are nonfunctional, it will be important for future studies to confirm their physiological relevance. In support of the translational capacity of the dendritic mRNAs identified in our study, we confirmed the dendritic presence of protein products of two of those mRNAs. Notably, these two mRNAs, Hist1h4j and Med8 , encode proteins whose only known functions are in the nucleus. It will be of interest to investigate whether these proteins have a novel function within the dendrite, or translocate to the nucleus to exert their traditionally known function similar to other transcriptional regulators [29] , [34] . We found that many dendritic mRNAs rapidly associate with ribosomes in vivo after a novel experience. Though this was widely assumed to occur based on several lines of convergent data, it had never been directly tested. Rapid activity-induced increases in synaptic and dendritic translation have been observed in vitro in synaptoneurosome preparations [15] , [16] and cultured neurons [17] , [18] , [19] , [20] , [21] , with increased mRNA translation starting between 1–15 min after stimulation. These in vitro time courses are in agreement with the increased ribosome association observed in our in vivo study immediately after a 500-s novel experience. The relevance of rapid increases in dendritic translation for synaptic plasticity has been demonstrated in vitro [35] , [36] , [37] . In contrast, though previous in vivo studies have shown the general importance of translation for the formation of contextual fear memories and other types of memories [38] , [39] , these studies did not directly address the specific role of dendritic translation. Though our study does not directly measure translation of dendritic mRNAs, it does provide in vivo evidence for experience-regulated increases in ribosome association with dendritic mRNAs. Since it is likely that increased ribosome binding has a positive impact on mRNA translation and protein synthesis [40] , our data are in agreement with the widely assumed role of rapid dendritic protein synthesis in memory formation triggered by a novel experience. The results of our study provide additional experimental support for an important theoretical model of memory formation. This model, called the synaptic tagging model, is widely used to explain how learning can trigger the synapse-specific changes that are required to store new information within a neural circuit [41] , [42] . The synaptic tagging model proposes that an activated synapse adopts a protein synthesis-independent ‘tagged’ state that enables the synapse to capture ‘plasticity-related products’ (PRPs) such as mRNAs that are translated in dendrites and proteins that are synthesized in the soma. The model predicts that the recruitment of these PRPs to the tagged synapse stabilizes structural and functional changes within the tagged synapse, thereby enabling the long-term storage of memories. Neighbouring synapses that are not activated do not adopt a tagged state, and will as a result not capture the PRPs needed for stable change. However, the precise nature of the PRPs is unknown. Our data suggest the occurrence of a rapid first round of dendritic PRP synthesis that is enriched for proteins involved in cytoskeleton remodelling and translational machinery ( Fig. 5b ). Cytoskeletal remodelling seems to be an obvious early requirement for stabilizing structural changes in activated synapses. In parallel, rapidly synthesized translational machinery could be specifically recruited to tagged synapses, where it executes the synapse-specific synthesis of a putative second round of PRPs that further stabilize both structural and functional changes within tagged synapses [3] , [36] . It will be of great interest to apply our method for collecting ribosome-bound dendritic mRNA at later time-points after a novel experience in an attempt to identify the specific nature of this putative second round of PRPs. In addition, future studies could include additional experimental groups such as no-shock and immediate-shock groups to determine which PRPs might be specifically involved in contextual fear memory storage [43] . In summary, we developed the first method for collecting in vivo ribosome-bound dendritic mRNA, and used it for the first genome-wide characterization of experience-induced functional regulation of dendritic mRNAs. This revealed an unexpected breadth of dendritic mRNAs that bind to ribosomes after a brief novel experience, thereby supporting a model of synaptic plasticity that engages translation of a large variety of dendritically localized mRNAs. Future studies can use our method to identify, with high temporal resolution, all the dendritic mRNAs that undergo increased ribosome association upon any behavioural, pharmacological, genetic or other type of manipulation. Importantly, our method can be expanded to non-mouse models by using virus-mediated expression of EGFP-L10a under a Camk2a promoter or other promoter that can drive specific expression in neurons with a laminar organization. We anticipate that our method will be applied to animal models for a variety of brain disorders, thereby shedding light on the contribution of altered dendritic protein synthesis to brain pathophysiology. Transgenic animal creation All animal procedures were performed in accordance with the National Institutes of Health Guide for the Care and Use of Laboratory Animals and were approved by the Tufts University Institutional Animal Care and Use Committee. To create the tetO-EGFP-L10a transgenic mice, the CDS from an EGFP-L10a plasmid (gift from Nathaniel Heintz, Rockefeller University) was cloned into an EcoRV site in pMM400Sfi (gift from Mark Mayford, The Scripps Research Institute) with blunt ligation to create a tetO-EGFP-L10a construct. Pronuclear microinjection into C57BL/6J embryos was performed at the Tufts Medical Center Transgenic Core Facility. Several transgenic founder lines were screened for expression levels of EGFP-L10a after breeding with Camk2a-tTA transgenic mice. One line with strong, specific expression was used for all further experiments (JAX Stock Number 024898). Fear conditioning Male and female, 2–3-month-old heterozygous Camk2a-tTA/tetO-EGFP-L10a mice on a C57BL/6J background were singly housed and either left in their cage until tissue dissection or submitted to a single contextual fear conditioning trial. Fear conditioning trials were performed in a specialized chamber (H10-11RTC, 120W × 100D × 120H; Coulbourn Instruments) and consisted of 500 s with 2 s, 0.7 mA foot shocks administered at 198, 278, 358 and 438 s. Freezing behaviour was measured using a digital camera connected to a computer with Actimetrics FreezeFrame software. Before-shock freezing scores were obtained by averaging freezing during 2 and 3 min of the trial. After-shock freezing scores were obtained by averaging freezing during the final 40 s of the trial. Tissue dissection Immediately after the fear conditioning trial or after removal from the home cage, the mice were anesthetized with isoflurane. The brain was rapidly removed in an ice cold dissection buffer (1 × HBSS, 2.5 mM HEPES-KOH, 35 mM glucose, 4 mM NaHCO3) and then frozen in liquid nitrogen. Coronal sections (~0.5 mm thick) were manually cut using a sterile scalpel and the brain slices were kept frozen in RNase-free 60% glycerol cooled to −10 °C using a cold plate (TCP-2D, Thermoelectrics Unlimited). Tissue punches of CA1 soma or dendrites were collected under a dissection scope with a 30-gauge blunt needle (Hamilton 7762-03). Individual tissue punches were placed in 50-μl homogenization buffer [12] , frozen in liquid nitrogen and stored at −80 °C until RNA isolation. Each brain slice was placed in 4% paraformaldehyde (PFA) overnight, moved to 30% sucrose for 1 day and then stained with 4',6-diamidino-2-phenylindole (DAPI). Brain slices were inspected on both sides to ensure accurate placement of each punch in the hippocampus. Dendritic punches were excluded if they touched the CA1 somatic layer at any point, ensuring no contamination with CA1 somatic RNA in any of the dendritic samples. Accurately placed dendritic or somatic tissue punches from individual mice were pooled before immunoprecipitation. RNA isolation RNA was isolated using a modified version of the Translating Ribosome Affinity Purification technique [12] , [13] that was optimized to remove background. Our method has lower background compared with the original method that uses magnetic beads linked to Protein G or Protein L to bind to two anti-GFP antibodies (bioreactor SN preparations of clones HtzGFP-19C8 and HtzGFP-19F7, 50 μg of each antibody) [12] , [13] , [44] as well as GFP-binding nanobodies linked to magnetic or agarose beads (ChromoTek) ( Supplementary Fig. 1c–f ). In our method a single anti-GFP antibody from the Monoclonal Antibody Core Facility at the Memorial Sloan-Kettering Cancer Center (purified form of HtzGFP-19C8, 10 μg antibody per mg magnetic beads) was covalently bound to magnetic epoxy beads (Invitrogen) followed by bovine serum albumin treatment to reduce nonspecific binding. Tissue samples were homogenized before being added to prepared beads. Samples were incubated with the beads for 1 h at 4 °C. The SN was saved for comparison to the IP. After five washes with a KCl buffer [12] , RNA was extracted with Trizol LS. A back extraction was used to improve yield. Organic contaminants were removed with butanol and water-saturated diethyl ether washes [45] . RNA was precipitated using NaOAc, isopropanol and linear acrylamide overnight at −80 °C. After two washes with 80% EtOH, the RNA was resuspended in 10-μl nuclease-free water. Concentration was measured using Ribogreen (Invitrogen). IP RNA yields were typically in the low hundreds of picograms range. Reverse transcription and qPCR Reverse transcription (RT) was performed with Superscript III (Invitrogen) according to the manufacturer’s instructions, except both random hexamers and anchored-oligo dT primers were used to prime the RT reaction. qPCR was performed with SYBR Green PCR Master Mix (Applied Biosystems) on either a Mx3000P or Mx4000 thermal cycler (Agilent). Library preparation and sequencing RNA was amplified and converted to complementary DNA using the Ovation RNA-Seq V2 Kit (Nugen) according to the manufacturer’s instructions. The Ovation RNA-Seq kit utilizes custom oligo dT and random primers that do not bind to ribosomal sequences during RT and work well on fragmented samples [46] . Excess single-stranded DNA products were removed using Promega S1 nuclease [47] . Libraries were prepared using the TruSeq DNA Sample Preparation v2 Kit (Illumina). PCR cycles were titrated to ensure minimal amplification bias. Size selection was performed using SizeSelect E-Gels (Invitrogen). Finished libraries were sequenced on the HiSeq2000 at the Tufts University Core Facility. Libraries at ~300 bp (~180-bp insert size) were used for 50 bp single end sequencing and libraries at ~400 bp (~280 bp insert size) were used for 100 bp paired end sequencing. Read alignment and quantification Sequencing quality control was performed using FastQC (Barbraham Institute). Reads were aligned using STAR (version 2.1.1d) [48] . Unique read counts per gene were determined using HTSeq (version 0.5.4p3) [49] and used for intersample comparisons. Clustering analysis was performed on count data using variance stabilizing transformation as part of the DESeq R package [50] . To allow for intrasample comparison of gene expression, we used Cufflinks (version 2.0.2) [51] to generate normalized FPKM read values with ribosomal and mitochondrial sequences masked. Custom gene annotations were created based on the mm9 UCSC annotation. Each gene was split into a CDS(+) portion containing the 5′UTR, CDS and 0, 50, 100, 150, 200, 250 or 300 bp of the 3′UTR and a 3′UTR (−) portion containing the remaining 3′UTR. Cufflinks quantification was performed separately with each of the resulting genome annotations as well as with an unaltered genome annotation and one containing only CDS. Curation of control gene lists To verify the success of EGFP-L10a immunoprecipitation in collecting mRNA from dendrites of CA1 pyramidal neurons, we curated two lists of control genes: genes that within the CA1 region of the hippocampus are only expressed within the excitatory pyramidal neurons (+pyr), and genes that within the CA1 are only expressed outside of the pyramidal neurons (−pyr). Initial lists of potential +pyr and –pyr genes were generated from previous transcriptome and in situ [8] , [52] , [53] studies, as well as the Neuroblast and fine structure search functions on the Allen Mouse Brain Atlas [25] ( Supplementary Data 1 ). Each of the 1,238 genes in these initial lists were manually inspected on the Allen Mouse Brain Atlas and the Brain Gene Expression Map [54] to confirm specific expression within or outside of CA1 pyramidal neurons. This yielded final lists of 74 +pyr genes and 124 −pyr genes ( Supplementary Data 1 ). Application of machine learning We used supervised, binary machine learning classification to predict which genes were ribosome bound in dendrites and soma. Each gene had four expression values (IP CDS(+), SN CDS(+), IP 3′UTR(−) and SN 3′UTR(−)) in all data sets except the unaltered annotation and CDS-only annotation, which only had expression values for IP and SN. The lists of +pyr and –pyr genes were used as training examples for the algorithm after filtering out those with low expression (all FPKM values<1). In the case of the somatic sample, +pyr genes with IP/SN ratios<1 were also removed. We reasoned that these represented transcripts that were present in the cells but not bound to ribosomes. Classification was achieved with a linear SVM algorithm using the e1071 R package. Cost was determined by training for the optimal k-1 fold cross validation. Receiver operating characteristic (ROC) curves were generated using the ROCR R package [55] . Supplementary Data 2 and 3 report all genes in the dendritic and somatic lists along with their FPKM values, classification results and the SVM distance. The SVM distance is a measure of the distance between the gene data points and the maximally-separating hyperplane constructed by the SVM algorithm. Genes with a positive distance were classified as being bound to ribosomes in the dendrite/soma (Y) and genes with a negative distance were classified as not being bound to ribosomes in the dendrite/soma (N). GO analysis was performed using DAVID (david.abcc.ncifcrf.gov) [56] , [57] . Immunohistochemistry To prepare brain tissue for IHC, Thy1–YFP [26] or C57BL/6 mice were anesthetized with ketamine/xylazine and transcardially perfused with 0.1 M Phosphate Buffer (PB) followed by 4% PFA in 0.1 M PB. Brains were extracted and post fixed in 4% PFA for 24 h. Brains were transferred to 30% sucrose for 48–72 h before being frozen. Coronal sections were sliced at 20 μm using a cryostat. Sections were stored in cryoprotectant at −20 °C until used. Sections were rinsed in Phosphate-Buffered Saline (PBS) with 0.25% Triton X-100 (PBS-T). Sections were then blocked for 1 h at room temperature in PBS-T with a 10% normal donkey or goat serum. Primary antibodies (Abcam rabbit anti-histone H4 1/100, Santa Cruz goat anti-Med8 1/50, Millipore mouse anti-Gad1 1/10,000 and Aves chicken anti-GFP 1/500) were diluted in the blocking solution, incubated overnight at 4 °C and rinsed three times for 15 min in PBS-T. Secondary antibodies (all from Jackson Immuno Research; goat anti-rabbit Cy3 1/2,000, goat anti-mouse Cy3 1/2,000, donkey anti-rabbit 647 1/1,000 and goat anti-chicken 488 1/500) were diluted in the blocking solution and were then applied to the sections for 2 h at room temperature followed by three rinses for 15 min in PBS-T. Sections were stained with DAPI to label cell nuclei, mounted on slides and coverslipped before being stored at 4 °C until imaged. In-situ probe creation The following primers were used to create in situ probes using whole hippocampus complementary DNA as a template: Pafah1b1: forward 5′-AAAATGGTGCTGTCCCAGAG-3′ and reverse 5′-ACACGGAGGGTCTTGTCATC-3′, Med8: forward 5′-GACCTGGCCCTCTGTCCT-3′ and reverse 5′-CTTGCCGAAAGCCTGTGT-3′, Hist1h4j: forward 5′-TCATGTCTGGCAGAGGTAAGG-3′ and reverse 5′-TTGCATCCGAGACAGCATAG-3′. Primers were designed using Primer 3 (ref. 58 ). PCR products were cloned into pCRII-TOPO using the TOPO TA Cloning Kit (Invitrogen). Insert sequences were verified with Sanger sequencing. Based on insert orientation, NotI or SpeI restriction endonucleases (NEB) were used to linearize the vector prior to in vitro transcription. Probes were synthesized using digoxigenin-11-UTP (Roche) and T7 or SP6 RNA Polymerase (NEB) according to the manufacturer’s instructions. Template DNA was removed with TURBO DNase (Applied Biosystems) according to the manufacturer’s instructions. FISH Dual FISH and IHC labelling was performed as previously described [59] on Thy1–YFP mice that were perfused immediately after contextual fear conditioning. Fear conditioning was used because neuronal activation has been reported to release dendritic mRNA from RNA-binding complexes, thereby facilitating in situ detection of the mRNA [21] . Brain tissue was prepared as detailed in the Immunohistochemistry section, but under RNase-free conditions. Selected 20-μm brain sections were mounted on HistoBond slides (VWR), desiccated overnight at 42 °C, washed in diethylpyrocarbonate (DEPC)-PBS and then incubated in a proteinase K wash (50 mM Tris pH 8.0, 25 mM EDTA, 160 ml DEPC-dH20, 200 μg proteinase K) for 30 min at 37 °C. The slides were washed again in DEPC-PBS and transferred to 0.25% acetic anhydride in 0.1 M triethanolamine for 10 min. Sections were briefly washed in DEPC-PBS and dried at room temperature. The hybridization was performed overnight at 52 °C using a humidified, temperature controlled chamber (Boekel Slide Moat Model #240000) in hybridization buffer (50% formamide, 2 × SSC, 1 × Denhart’s solution, 0.25 M Tris pH 8.0, 10 mM DTT, 0.5% SDS, 10% dextran sulphate and 265 μg ml −1 salmon sperm DNA) containing the digoxigenin-labelled probe diluted at a ratio of 1:50. Slides were washed in 1 × SSC, treated with RNase A (Sigma) for 1 h at 37 °C, washed with 1 × SSC followed by 0.5 × SSC at room temperature and then washed three times with 0.1 × SSC at 65 °C. Tissue was prepared for labelling by incubating for 15 min at room temperature in 0.5% hydrogen peroxide and 0.5% Triton X in PBS. Slides were then washed three times in PBS. After a 10 min incubation in maleic acid buffer (100 mM maleic acid, 150 mM NaCl, pH 7.5) at room temperature, tissue was blocked for 10 min at room temperature in 1% blocking solution (Roche). Primary antibody (Roche anti-digoxigenin-POD 1:100, Invitrogen Rabbit Anti-GFP 1:2,000) incubation was performed overnight at 4 °C in 1% blocking solution. After three 10 min washes in PBS, the slides were incubated 30 min at room temperature in a biotinylated tyramide solution consisting of 8.25% hydrogen peroxide in PBS (biotinylated tyramide prepared according to Perkin Elmer TSA Biotin kit instructions). After a 30 min incubation at room temperature, slides were washed three times for 10 min in PBS at room temperature. Secondary antibody (Invitrogen Alexa-Strep-488 1:500, Jackson Immuno Research Cy3-AffiniPure Goat Anti-Rabbit IgG 1:2,000) incubation was performed for 2 h at room temperature in 1% blocking solution. Slides were washed in PBS for 10 min, dried and then mounted with ProLong Gold with DAPI (Life Technologies). Image collection and analysis A confocal laser-scanning microscope was used for all image acquisition (Nikon A1R) except Fig. 1f where a widefield epifluorescence microscope was used (Nikon E800) and Fig. 1b where a slide scanner was used (Zeiss Axio Imager Z2 epifluorescence microscope with a Maerzhaeuser motorized scanning stage). When imaging sense and antisense in situ probes, the settings for PMT, laser power, gain and offset were identical. Images were analyzed using the NIS Elements Viewer v4.0. The same lookup-table settings were used for the sense and antisense probe images. Accession codes: The data discussed in this publication have been deposited in NCBI's Gene Expression Omnibus [60] and are accessible under GEO Series accession number GSE58343 How to cite this article: Ainsley, J. et al. Functionally diverse dendritic mRNAs rapidly associate with ribosomes following a novel experience. Nat. Commun. 5:4510 doi: 10.1038/ncomms5510 (2014).